mRNA 3′-UTR shortening is a molecular signature of mTORC1 activation Mammalian target of rapamycin (mTOR) enhances translation from a subset of messenger RNAs containing distinct 5′-untranslated region (UTR) sequence features. Here we identify 3′-UTR shortening of mRNAs as an additional molecular signature of mTOR activation and show that 3′-UTR shortening enhances the translation of specific mRNAs. Using genetic or chemical modulations of mTOR activity in cells or mouse tissues, we show that cellular mTOR activity is crucial for 3′-UTR shortening. Although long 3′-UTR-containing transcripts minimally contribute to translation, 3-′UTR-shortened transcripts efficiently form polysomes in the mTOR-activated cells, leading to increased protein production. Strikingly, selected E2 and E3 components of ubiquitin ligase complexes are enriched by this mechanism, resulting in elevated levels of protein ubiquitination on mTOR activation. Together, these findings identify a previously uncharacterized role for mTOR in the selective regulation of protein synthesis by modulating 3′-UTR length of mRNAs. In eukaryotes, a large portion of mRNAs contains multiple polyadenylation signals (PASs) in their 3′-untranslated region (3′-UTR). Alternating the usage of PAS, namely alternative cleavage and polyadenylation (ApA), produces mRNA isoforms with the same coding capacity but with various lengths of 3′-UTR [1] , [2] , [3] , [4] . As 3′-UTR provides a binding platform for microRNAs and RNA-binding proteins, it serves as an important determinant for mRNA fate such as translation and stability [2] , [3] , [5] , [6] . Therefore, ApA provides an additional layer of complexity in regulating gene expression at the posttranscriptional level. Powerful high-profiling technologies focusing on 3′-UTRs of mRNAs provided high-resolution snap shots of alternatively polyadenylated mRNA isoforms in various tissues and cells across many species [6] , [7] , [8] , [9] , [10] , [11] . An important insight that emerged from these studies is that 3′-UTR length undergoes dynamic changes under pathogenic conditions such as cancer and in diverse biological processes such as cell proliferation, differentiation and development [2] , [6] , [7] , [12] , [13] , [14] . Although the information on alternative polyadenylation sites in transcriptomes across different species and tissues is rapidly accumulating, it is not clear what cellular mechanism(s) controls the switches between proximal and distal polyadenylation sites and how this process is regulated. The mammalian target of rapamycin (mTOR) pathway is crucial for regulating cell proliferation/growth and its dysregulation causes many human diseases [15] . mTOR exists as two distinctive multi-protein complexes, mTORC1 and mTORC2. Raptor and Rictor are specific components of mTORC1 and mTORC2, respectively, and they are essential for cellular function of each mTOR complex [15] , [16] . mTORC1 is negatively regulated by tuberous sclerosis complexes (TSC1 and TSC2) and is an evolutionarily conserved kinase that phosphorylates the ribosomal protein S6 kinases and the eukaryotic initiation factor 4E-binding proteins for efficient translation [15] , [16] . Recent studies identified cis -acting elements in mRNAs such as 5′-terminal oligopyrimidine tract (TOP) or 5′-pyrimidine-rich translational element (PRTE) that render the association of a transcript with polysomes. mRNAs containing these elements in their 5′-UTRs encode proteins for cellular pathways including translation, cell invasion and metastasis, suggesting their relevance in cancer pathogenesis [17] , [18] . mTOR also plays an important role for activating transcriptional networks and regulates multiple cellular pathways for lipid and nucleotide metabolism [19] , [20] . Recently, mTOR was shown to play a role in the regulation of proteasome activity by upregulating a transcription factor Nrf-1 (ref. 21 ). Although these studies were mainly focusing on the role of mTOR in the synthesis of proteins, lipids and nucleic acids through transcriptional networks, whether mTOR is involved in other cellular processes by modulating gene expression at posttranscriptional level is relatively unclear. In this study, we used isogenic non-cancerous mouse embryonic fibroblast (MEF) cell lines to understand changes of molecular features on dysregulated activation of mTOR. We employed RNA sequencing (RNA-seq) and two-dimensional liquid chromatography tandem mass spectrometry (2D LC–MS/MS) approaches to investigate the changes at high resolution and found an unexpected link between mTOR and ubiquitin-mediated proteolysis pathway through 3′-UTR shortening. These findings expand our understanding of mTOR to regulation of RNA processing and protein degradation pathways. 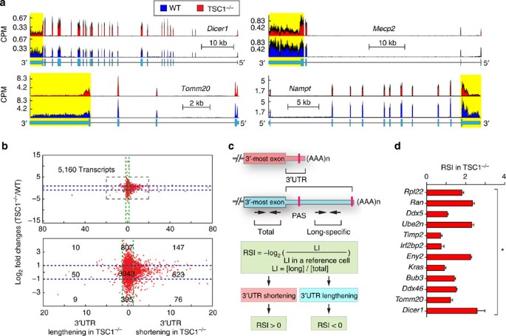Figure 1: mTOR activation leads to genome-wide 3′-UTR shortening. (a) RNA-seq reads from WT and TSC1−/−are aligned to mouse genome mm10 RefSeq. Representative examples of transcripts with 3′-UTR shortening are presented. Annotated gene structures are at the bottom of the alignment. The yellow boxes highlight the aligned reads in 3′-UTRs. (b) Scatter plot of RNA-seq data. Red dots represent individual transcripts in the analysis. Horizontal blue-dashed lines represent the cutoff values for twofold changes in differential gene expression. Vertical green-dashed lines represent the cutoff values for −log10(P-value) of 3′-UTR shortening (1.3 corresponds toP=0.05) in TSC1−/−and WT, which was determined byχ2-test. (c) A schematic presenting primer sets for RT–qPCR and the RSI determination. Pairs of primers were used to detect a total (short+long) or a long-specific transcript. The RSI was calculated to determine the 3′-UTR shortening in a target cell line by RT–qPCR. (d) Validation of RNA-seq data. Error bars represent s.e. from three repeats of experiments. Student’st-tests are done for statistical significance. *P<0.0025. mTOR activation leads to 3'-UTR shortening of mRNAs To explore mTOR function in gene expression at a single nucleotide resolution, we performed RNA-seq experiments ( Supplementary Table 1 ) using Tsc1 knockout (TSC1 −/− ) and wild-type (WT) MEF cells [22] . Knockout of Tsc1 , a negative regulator of mTOR, leads to uncontrolled mTOR hyperactivation compared with WT [22] , [23] . One of the striking features in our data set was that many transcripts in TSC1 −/− showed an abrupt signal drop only for a segment of the 3′-most exon of an annotated gene compared with WT ( Fig. 1a and Supplementary Fig. 1a ). For example, the read signal for Dicer1 in TSC1 −/− dropped after the termination codon in the 3′-most exon, although the signal from upstream exons increased ( Fig. 1a ). In some cases, upstream exons showed either similar (for example, Mecp2 and Tomm20 ) or decreased (for example, Anxa7 and Timp2 ) signal, although we observed the same pattern of signal drop in the 3′-most exon from TSC1 −/− ( Fig. 1a and Supplementary Fig. 1a ). Further sequence analysis revealed that canonical or non-canonical PAS(s) exists around the regions showing the signal drop. This indicates that the synthesis of these transcripts terminated early in the 3′-most exon using the proximal PASs for polyadenylation, suggesting a predominant production of mRNA isoforms with a shorter 3′-UTR in the mTOR-activated transcriptome ( Fig. 1a and Supplementary Fig. 1a , yellow box, and Supplementary Data 1 ). For some transcripts such as Tomm20 and Nampt , 3′-UTR-shortened transcripts were already present in WT where the mTOR activity is low but not entirely absent ( Fig. 1a and Supplementary Fig. 1a ). These 3′-UTR-shortened transcripts increased significantly in TSC1 −/− ( Fig. 1a and Supplementary Fig. 1a ), indicating that individual transcripts differ in the regulation of their 3′-UTR length in response to cellular mTOR activity. As the signals from upstream exons reflecting the amount of transcripts varied among the 3′-UTR-shortened transcripts, we examined whether 3′-UTR shortening in the mTOR-activated transcriptome correlates to differential gene expression. To this end, we enriched 5,160 transcripts in our data set that are eligible for combined analysis of 3′-UTR shortening and differential expression (see Methods for details). Next, each transcript was plotted by fold changes in the differential gene expression ( y axis in Fig. 1b ) and the significance of 3′-UTR shortening ( x axis in Fig. 1b ). This approach identified 846 3′-UTR-shortened transcripts (about 16.4%) out of 5,160 transcripts in TSC1 −/− ( Fig. 1b ). Although 26.3% (223/846) of the 3′-UTR-shortened transcripts either increased (147/846) or decreased (76/846) their expression level, a significant proportion (73.7%) of them in the mTOR-activated transcriptome remained unchanged ( Fig. 1b ), indicating no strong correlation between the differential gene expression and the 3′-UTR shortening in the mTOR-activated transcriptome. Of note, only a small percentage (1.3%) of transcripts showed 3′-UTR shortening in WT over TSC1 −/− MEFs. To confirm the RNA-seq data, we developed a method to determine 3′-UTR shortening or lengthening by calculating ‘relative shortening index (RSI)’ (see Methods for details; Fig. 1c ). Twelve genes, covering a wide range of P -values, were randomly selected from the 3′-UTR shortening data set; all showed the RSI >0 in TSCI −/− ( Fig. 1d and see also Supplementary Fig. 1d,e for alternative presentations of the data using different experimental and calculation methods), validating our RNA-seq data analysis. Together, these data strongly suggest that mTOR activation in cells leads to a preferred usage of proximal PAS in the 3′-most exon of mRNAs and results in transcriptome-wide 3′-UTR shortening. Figure 1: mTOR activation leads to genome-wide 3′-UTR shortening. ( a ) RNA-seq reads from WT and TSC1 −/− are aligned to mouse genome mm10 RefSeq. Representative examples of transcripts with 3′-UTR shortening are presented. Annotated gene structures are at the bottom of the alignment. The yellow boxes highlight the aligned reads in 3′-UTRs. ( b ) Scatter plot of RNA-seq data. Red dots represent individual transcripts in the analysis. Horizontal blue-dashed lines represent the cutoff values for twofold changes in differential gene expression. Vertical green-dashed lines represent the cutoff values for −log 10 ( P -value) of 3′-UTR shortening (1.3 corresponds to P =0.05) in TSC1 −/− and WT, which was determined by χ 2 -test. ( c ) A schematic presenting primer sets for RT–qPCR and the RSI determination. Pairs of primers were used to detect a total (short+long) or a long-specific transcript. The RSI was calculated to determine the 3′-UTR shortening in a target cell line by RT–qPCR. ( d ) Validation of RNA-seq data. Error bars represent s.e. from three repeats of experiments. Student’s t -tests are done for statistical significance. * P <0.0025. Full size image 3′-UTR shortening is a downstream target of mTORC1 To determine whether 3′-UTR shortening due to ApA is a previously uncharacterized cellular target downstream of mTOR pathway, we established a stable mTOR knockdown cell line TSC1 −/− MEFs (TSC1 −/− mTOR kd; Supplementary Fig. 2a ). The tested transcripts showed the RSI <0 in TSC1 −/− mTOR kd MEFs as compared with a control knockdown cell line, indicating the enrichment of 3′-UTR-lengthened transcripts in mTOR-deficient cells ( Fig. 2a and Supplementary Fig. 2b ), thus supporting the idea that mTOR functions in 3′-UTR length regulation. Consistently, the same results were observed in a HEK293 stable cell line with mTOR knockdown or in a bladder cancer cell line HCV29 (where TSC1 is mutated and as a consequence, mTOR activity is upregulated) with TSC1 added back (HCV29 Add back) [24] , [25] . These results suggest that the function of mTOR in 3′-UTR shortening is a general phenomenon and evolutionarily conserved between human and mouse ( Supplementary Fig. 2c–e ). 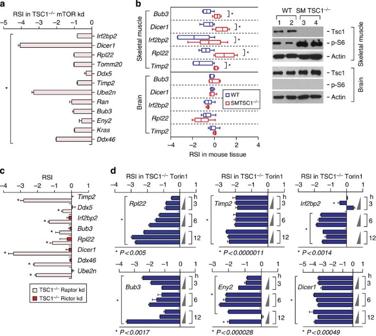Figure 2: 3′-UTR shortening is a downstream target of mTORC1. (a) mTOR knockdown (kd) in TSC1−/−recovers the 3′-UTR length. The RSI was measured using total RNAs isolated from TSC1−/−MEFs with mTOR kd. *P<0.015. (b) Activation of mTOR in terminally differentiated skeletal muscle leads to 3′-UTR shortening. Total RNAs from skeletal muscles in WT or skeletal muscle-specific knockout ofTsc1(SM TSC1−/−) mice were used for the RSI measurement. The brain was used as an additional tissue control. Western blotting on tissue extracts from two randomly chosen mice was done. p-S6 denotes phosphorylated S6, a downstream target of activated mTOR kinase. *P<0.016. (c) mTORC1 but not mTORC2 is crucial for 3′-UTR shortening. mTORC1 or mTORC2 was specifically deactivated by targeting Raptor or Rictor, respectively, using short hairpin RNAs in TSC1−/−MEFs. The RSI was measured using RT–qPCR. *P<0.05. (d) A selective inhibitor of mTOR, Torin1, alters 3′-UTR length in mRNAs. TSC1−/−MEFs were treated with Torin1 at various doses (10, 50 and 250 nM, presented as incremental triangles) and time courses (3, 6 and 12 h). Changes in the 3′-UTR length were determined by measuring the RSI. *The conditions that accumulate the long 3′-UTR-containing transcripts with statistical significance. Figure 2: 3′-UTR shortening is a downstream target of mTORC1. ( a ) mTOR knockdown (kd) in TSC1 −/− recovers the 3′-UTR length. The RSI was measured using total RNAs isolated from TSC1 −/− MEFs with mTOR kd. * P <0.015. ( b ) Activation of mTOR in terminally differentiated skeletal muscle leads to 3′-UTR shortening. Total RNAs from skeletal muscles in WT or skeletal muscle-specific knockout of Tsc1 (SM TSC1 −/− ) mice were used for the RSI measurement. The brain was used as an additional tissue control. Western blotting on tissue extracts from two randomly chosen mice was done. p-S6 denotes phosphorylated S6, a downstream target of activated mTOR kinase. * P <0.016. ( c ) mTORC1 but not mTORC2 is crucial for 3′-UTR shortening. mTORC1 or mTORC2 was specifically deactivated by targeting Raptor or Rictor, respectively, using short hairpin RNAs in TSC1 −/− MEFs. The RSI was measured using RT–qPCR. * P <0.05. ( d ) A selective inhibitor of mTOR, Torin1, alters 3′-UTR length in mRNAs. TSC1 −/− MEFs were treated with Torin1 at various doses (10, 50 and 250 nM, presented as incremental triangles) and time courses (3, 6 and 12 h). Changes in the 3′-UTR length were determined by measuring the RSI. *The conditions that accumulate the long 3′-UTR-containing transcripts with statistical significance. Full size image Proliferative cells are known to carry short 3′-UTRs in their transcriptome and terminally differentiated tissues are known to produce transcripts with long 3′-UTRs [6] , [7] , [10] . We asked whether mTOR activation could be an underlying reason that explains these observations. We used a mouse model with skeletal muscle-specific Tsc1 knockout (SM TSC1 −/− ) to render mTOR hyperactivated only in skeletal muscle ( Fig. 2b and Supplementary Fig. 2f ) [26] and compared the changes in 3′-UTR length. Control brain tissues from both WT and SM TSC1 −/− did not show significant changes in 3′-UTR length ( Fig. 2b ). In contrast, the RSI of the tested transcripts in the skeletal muscle from SM TSC1 −/− mice was >0 as compared with that from WT, providing evidence that the mTOR activation is sufficient to drive 3′-UTR shortening in terminally differentiated skeletal muscles ( Fig. 2b and Supplementary Fig. 2m ). To address which mTOR complex regulates 3′-UTR shortening, we established stable cell lines using short hairpin RNA that specifically knocks down Raptor (a component of mTORC1) or Rictor (a component of mTORC2) in TSC1 −/− MEFs ( Supplementary Fig. 2g ). The knockdown of Raptor but not Rictor resulted in the RSI <0 when compared with control knockdown cells, suggesting that mTORC1 plays an important role in 3′-UTR shortening ( Fig. 2c and Supplementary Fig. 2h ). mTOR is a key therapeutic target for many human disease treatments [15] and several versions of selective mTOR inhibitors have been developed including Torin1 (ref. 27 ). Thus, we examined whether pharmacological inhibition of mTOR via Torin1 could modulate ApA. Torin1 treatment of TSC1 −/− or HEK293 cells resulted in the RSI <0 in most of the tested transcripts in all conditions and the lengthening of 3′-UTR occurred as early as 3 h after the treatment, indicating that the cellular ApA pattern changes drastically on the inhibition of mTOR ( Fig. 2d and Supplementary Fig. 2i,j,n ). In contrast, the treatment of rapamycin, which does not fully inhibit mTORC1 (refs 18 , 28 ) showed minimal effect, if any, on 3′-UTR lengthening ( Supplementary Fig. 2j–l ). As Torin1 arrests cells in G1/S phase [27] , [28] , the lengthening of the 3′-UTR on Torin1 treatment could come from the inhibition of cell proliferation. To rule out this possibility, we used another class of small molecules such as hydroxyurea or mimosine, which arrest cells in G1/S without downregulating mTOR activity ( Supplementary Fig. 2o ) [29] , [30] . Hydroxyurea or mimosine treatment for 12 h in WT MEFs showed the RSI >0, indicating that 3′-UTR shortening occurred even though cells stop proliferating ( Supplementary Fig. 2p ). However, the same treatment of WT MEFs with mTOR knockdown abolished 3′-UTR shortening ( Supplementary Fig. 2q ). Thus, the 3′-UTR lengthening after Torin1 treatment is not caused by the inhibition of cell proliferation but rather from the inactivation of mTOR ( Supplementary Fig. 2r,s ). Taken together, we conclude that the mTOR pathway is an upstream regulator for ApA process and determines the 3′-UTR length in the transcriptome independent of cell proliferation status. 3′-UTR shortening activates ubiquitin-mediated proteolysis Activation of mTOR increases global protein synthesis by controlling multiple downstream events such as ribosome biogenesis and cap-dependent translation initiation and elongation [15] , [16] . Especially, mTOR promotes the translation of a subset of mRNAs carrying 5′-UTR sequences such as 5′TOP, 5′TOP-like motif and 5′PRTE [17] , [18] . Similar to 5′-UTR, 3′-UTR in mRNA also plays an important role in the regulation of gene expression. In particular, 3′-UTR shortening in a transcript has been shown to increase protein production [3] , [6] , [7] , [31] . Therefore, we asked whether the mTOR-activated 3′-UTR shortening contributes to mTOR-mediated upregulation of protein synthesis and influences mTOR-related biology. To this end, we first conducted quantitative proteomic studies using tandem mass tag (TMT)-labelled total cell lysates prepared from WT and TSC1 −/− MEFs, to quantitatively profile the changes in the cellular proteome due to mTOR activation. We identified a total of 2,754 proteins that were found in either cell line by two or more unique peptides via 2D LC–MS/MS ( Supplementary Data 2 ). The KEGG (Kyoto Encyclopedia of Genes and Genomes) enrichment analysis on the catalogue of proteins with >20% increase (1,014 proteins) in abundance (TSC1 −/− compared with WT) shows that multiple cellular pathways are activated in TSC1 −/− ( Fig. 3a ). We also performed the KEGG pathway analysis using the catalogue of 846 3′-UTR-shortened transcripts ( Supplementary Data 1 ) and the differentially expressed transcripts in TSC1 −/− MEFs ( Supplementary Fig. 3a and Supplementary Data 3 ). By comparing the enriched pathways from these three data sets, we found that multiple pathways in the mTOR-activated proteome such as spliceosome (mmu03040) and RNA degradation (mmu03018) are upregulated by both 3′-UTR shortening and differential gene expression, whereas other enriched pathways such as DNA replication (mmu03030) and pyrimidine/purine metabolism (mmu00240/mmu00230) are attributable solely to the differential gene expression ( Fig. 3a and Supplementary Fig. 3a,b ). 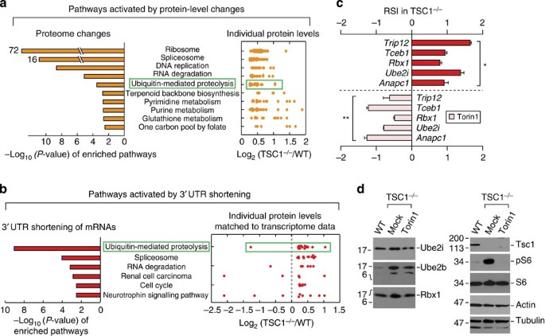Figure 3: 3′-UTR shortening due to mTOR activation targets specific cellular pathways including ubiquitin-mediated proteolysis. (a) Analysis of mTOR-activated proteome. The KEGG pathway enrichment analysis was performed using the catalogue of identified proteins from 2D LC–MS/MS. The left panel shows the enriched pathways in −log10(P-value). The right box shows the distribution of individual proteins in each KEGG pathway index shown in the left panel. Proteins showing more than 1.2 fold changes in TSC1−/−compared with WT MEFs are plotted. Ubiquitin-mediated proteolysis pathway is marked with a light green box. (b) Analysis of enriched KEGG pathways by 3′-UTR shortening in TSC1−/−MEFs. The mTOR-activated transcriptome is described inFigure 1. The KEGG pathways enriched in TSC1−/−MEFs by 3′-UTR shortening are shown in –log10(P-value). Fold changes of individual proteins in each pathway index are plotted in the right box. Ubiquitin-mediated proteolysis pathway is marked with a light green box. (c) The RSI was measured for the transcripts enriched in ubiquitin-mediated proteolysis pathway in TSC1−/−MEFs. The lengthening of 3′-UTR in TSC1−/−MEFs treated with Torin1 at 50 nM for 24 h was shown by the RSI. *P<1.5 × 10−6, **P<6.3 × 10−6. (d) Western blot analysis of E2 and E3 enzymes showing the 3′-UTR shortening in the RNA-seq experiments. Cells were treated with Torin1 for 24 h at 50 nM for 3′-UTR lengthening. pS6 denotes phosphorylated S6. Figure 3: 3′-UTR shortening due to mTOR activation targets specific cellular pathways including ubiquitin-mediated proteolysis. ( a ) Analysis of mTOR-activated proteome. The KEGG pathway enrichment analysis was performed using the catalogue of identified proteins from 2D LC–MS/MS. The left panel shows the enriched pathways in −log 10 ( P -value). The right box shows the distribution of individual proteins in each KEGG pathway index shown in the left panel. Proteins showing more than 1.2 fold changes in TSC1 −/− compared with WT MEFs are plotted. Ubiquitin-mediated proteolysis pathway is marked with a light green box. ( b ) Analysis of enriched KEGG pathways by 3′-UTR shortening in TSC1 −/− MEFs. The mTOR-activated transcriptome is described in Figure 1 . The KEGG pathways enriched in TSC1 −/− MEFs by 3′-UTR shortening are shown in –log 10 ( P -value). Fold changes of individual proteins in each pathway index are plotted in the right box. Ubiquitin-mediated proteolysis pathway is marked with a light green box. ( c ) The RSI was measured for the transcripts enriched in ubiquitin-mediated proteolysis pathway in TSC1 −/− MEFs. The lengthening of 3′-UTR in TSC1 −/− MEFs treated with Torin1 at 50 nM for 24 h was shown by the RSI. * P <1.5 × 10 −6 , ** P <6.3 × 10 −6 . ( d ) Western blot analysis of E2 and E3 enzymes showing the 3′-UTR shortening in the RNA-seq experiments. Cells were treated with Torin1 for 24 h at 50 nM for 3′-UTR lengthening. pS6 denotes phosphorylated S6. Full size image Intriguingly, among those enriched pathways in the quantitative proteome analysis, ribosome- (mmu03010) and ubiquitin-mediated proteolysis pathways (mmu04120) did not appear in the differential gene expression data set ( Fig. 3a and Supplementary Fig. 3b,c ). This indicates that these two pathways are most likely to be activated by other mTOR-mediated regulatory mechanisms rather than transcriptional regulation. It is known that the ribosome pathway is activated by mTOR through the translational regulation of mTOR-responsive 5′-UTR cis -elements such as 5′TOP and 5′PRTE in the mRNAs [17] , [18] , [32] . On the other hand, mTOR-responsive 5′-UTR sequence elements do not exist in most transcripts from the ubiquitin-mediated proteolysis pathway, supporting the idea that 3′-UTR shortening could be an explanation for the activation of ubiquitin-mediated proteolysis pathway in the mTOR-activated proteome (the light green box in Fig. 3a,b and Supplementary Fig. 3d ). All transcripts from the ubiquitin-mediated proteolysis pathway containing short 3′-UTR encode the components of E2 ubiquitin-conjugating enzymes and E3 ubiquitin ligases such as Anapc1 , Rbx1 , Trip12 , Ube2i and Tceb1 . Consistent with our findings in this study, these transcripts carry an mTOR-dependent short 3′-UTR in TSC1 −/− MEFs as determined by the RSI in the presence or the absence of Torin1 treatment ( Fig. 3c ). As shown by western blotting ( Fig. 3d ), the expression of Ube2i, Ube2b and Rbx1 proteins matched the progression of 3′-UTR shortening in these transcripts, supporting our conclusions from quantitative proteomics studies and 3′-UTR-shortening analysis. Together, these results suggest that 3′-UTR shortening by mTOR activation plays an important role in altering gene expression. These results also identify the ubiquitin-mediated proteolysis pathway as an additional cellular target of mTOR. Thus, mTOR-driven 3′-UTR shortening might explain part of cellular phenotypic changes in TSC1 −/− over WT MEFs. 3′-UTR shortening contributes to mTOR-promoted translation To examine whether 3′-UTR shortening in the group of transcripts of the ubiquitin-mediated proteolysis pathway is the major contributor to the increase in protein production, we looked at the effect of mTOR-mediated 3′-UTR shortening on the association with actively translating ribosomes using polysome fractionation and reverse transcription–quantitative PCR (RT–qPCR). We fractionated cytoplasmic extracts on sucrose gradients to separate polysomes from 40S, 60S and 80S (monosome) ribosomes ( Fig. 4a ). Using RT–qPCR on RNAs purified from each fraction, we measured the percentage of total (long+short) and long 3′-UTR transcripts (see the Supplementary Materials for details) in each tested cell line. Interestingly, an overall distribution of long 3′-UTR transcripts across the separated fractions was polarized into light (fractions 2 and 3) and heavy fractions (fractions 6, 7 and 8; Rbx1 , Ube2i , Anapc1 and Ube2n ) or was biased to light fractions (fractions 2 and 3; Trip12 and Tceb1 ) ( Fig. 4b and Supplementary Fig. 4a ). In cases of Rpl22 and Bub3 , long 3′-UTR transcripts were distributed almost evenly across the separated fractions ( Supplementary Fig. 4a ). All these results indicate that a significant portion of long 3′-UTR transcripts are not translated in cells or do not associate with ribosomes efficiently. In contrast, the overall distribution of total (long+short) transcripts was biased towards heavy polysome fractions (fractions 7 through 11) in all cell lines ( Fig. 4b and Supplementary Fig. 4a ). The association of total transcripts with polysomes was more prominent in TSC1 −/− compared with WT or TSC1 −/− treated with Torin1. As total transcripts contain both long and short 3′-UTR transcripts, we compared the distribution of short 3′-UTR transcripts with that of total. To do this, we first conducted rapid amplification of complementary DNA 3' ends to locate the precise proximal poly(A) sites of short 3′-UTR transcripts ( Supplementary Fig. 4e ) and used oligo d(T) 30 primers with 3′-end degenerated C (for Rbx1 ) or G (for Anapc1 ) for amplification. RT–PCR and agarose gel-based detection of total, short and long 3′-UTR transcripts for Rbx1 and Anapc1 in each fraction from TSC1 −/− revealed that most short 3′-UTR transcripts formed polysomes, whereas a significant fraction of long 3′-UTR transcripts do not ( Supplementary Fig. 4b ). These results are consistent with the observations made by RT–qPCR. Importantly, the distribution of total transcripts mirrors short 3′-UTR transcripts more than long 3′-UTR transcripts ( Supplementary Fig. 4b ). Thus, highly enriched total transcript signals in the polysome fractions of TSC1 −/− are likely to be due to the presence of short 3′-UTR transcripts. Considering the biggest differences between total and long transcript signals in the polysome fractions, short 3′-UTR transcripts are the major form of mRNAs in polysomes and determine protein synthesis in TSC1 −/− MEFs. Contrary to this, in WT MEFs the overall total transcript signals from the polysome fractions are reduced and the proportion of long 3′-UTR transcripts is close to that of total transcripts in polysomes ( Fig. 4b and Supplementary Fig. 4a ). Intriguingly, the distribution and percentage of long 3′-UTR-containing transcripts showed minimal, if any, changes in different cellular contexts (WT, TSC1 −/− and TSC1 −/− treated with Torin1; Fig. 4b and Supplementary Fig. 4a ). These results propose that long 3′-UTR transcripts participate in the basal level of protein synthesis regardless of cellular contexts and play a bigger role in translation in WT compared with TSC1 −/− . Together, these results provide evidence that short 3′-UTR transcripts define part of proteome changes on mTOR activation. We also noted that in the presence of 50 nM Torin1 for 24 h, formation of polysomes with total transcripts decreased, while formation of polysomes with long 3′-UTR transcripts stayed constant ( Fig. 4b and Supplementary Fig. 4a ). This suggests that the formation of polysomes in TSC1 −/− is largely dependent on the level of short 3′-UTR transcripts. 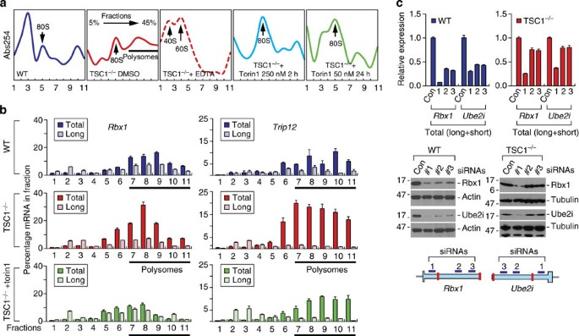Figure 4: 3′-UTR shortening is an mTORC1-activated molecular signature for protein synthesis. (a) Polysome fractionation using 5%–45% sucrose gradient. Cytoplasmic extracts were prepared from WT, TSC1−/−MEFs in the presence or the absence of 50 mM EDTA, or in the presence of 50 nM or 250 nM Torin1. Eleven fractions were collected and subjected to absorbance measurement at 254 nm. The arrows mark 40S, 60S subunits and 80S monosomes. The black thick line indicates polysome fractions (fractions 7 through 11). (b) Polysome analyses of selected total (long+short) and long transcripts in each fraction from sucrose gradient. Percentage of total and long transcripts forRbx1orTrip12in each fraction was measured using RT–qPCR. (c) Long 3′-UTR-containing transcripts minimally contribute to protein synthesis on mTOR activation. siRNAs targeting three distinct regions in the 3′-UTR ofRbx1andUbe2imRNAs were designed (right bottom panel). siRNA#1 targets the region between the termination codon and the first PAS. siRNAs#2 and 3 specifically targets long 3′-UTR-containing transcripts only. Knockdown of total or long transcripts was carried out using these siRNAs in WT and TSC1−/−MEFs. The amounts of remainingRbx1andUbe2itotal (long+short) transcripts were measured using RT–qPCR (left panel). Western blotting was performed using the cell lysates from RNA interference knockdown experiments (right top panel). Figure 4: 3′-UTR shortening is an mTORC1-activated molecular signature for protein synthesis. ( a ) Polysome fractionation using 5%–45% sucrose gradient. Cytoplasmic extracts were prepared from WT, TSC1 −/− MEFs in the presence or the absence of 50 mM EDTA, or in the presence of 50 nM or 250 nM Torin1. Eleven fractions were collected and subjected to absorbance measurement at 254 nm. The arrows mark 40S, 60S subunits and 80S monosomes. The black thick line indicates polysome fractions (fractions 7 through 11). ( b ) Polysome analyses of selected total (long+short) and long transcripts in each fraction from sucrose gradient. Percentage of total and long transcripts for Rbx1 or Trip12 in each fraction was measured using RT–qPCR. ( c ) Long 3′-UTR-containing transcripts minimally contribute to protein synthesis on mTOR activation. siRNAs targeting three distinct regions in the 3′-UTR of Rbx1 and Ube2i mRNAs were designed (right bottom panel). siRNA#1 targets the region between the termination codon and the first PAS. siRNAs#2 and 3 specifically targets long 3′-UTR-containing transcripts only. Knockdown of total or long transcripts was carried out using these siRNAs in WT and TSC1 −/− MEFs. The amounts of remaining Rbx1 and Ube2i total (long+short) transcripts were measured using RT–qPCR (left panel). Western blotting was performed using the cell lysates from RNA interference knockdown experiments (right top panel). Full size image To further investigate the effects of 3′-UTR shortening on protein synthesis in WT and TSC1 −/− MEFs, we designed small interfering RNAs (siRNAs) that target either total (siRNA 1) or long (siRNAs 2 and 3) 3′-UTR transcripts of Rbx1 and Ube2i specifically and measured their effects on gene expression by RT–qPCR and western blotting ( Fig. 4c ). Notably, siRNAs 2 and 3 minimally decreased total (long+short) mRNAs of Rbx1 and Ube2i in TSC1 −/− ( ∼ 20%–25% knockdown), whereas siRNA 1 could knock down those total mRNAs efficiently ( ∼ 60%–70%). On the other hand, siRNAs 2 and 3 increased the knockdown efficiency dramatically in WT (50–70%) compared with TSC1 −/− ( Fig. 4c ). As all siRNAs used in the experiment knocked down long 3′-UTR transcripts with high efficiency (70%–95%; Supplementary Fig. 4f ), the discrepancy in the efficiency of siRNAs 2 and 3 in WT and TSC1 −/− is likely to be due to the differences in the relative amounts of long 3′-UTR transcripts in these cells. The siRNA 1 significantly affected the protein levels of both Rbx1 and Ube2i in WT and TSC1 −/− . In contrast, the siRNAs 2 and 3 affected target protein levels only in WT ( Fig. 4c ). Taken together with polysome profiling experiments, these results suggest that most of the polysomes are formed with short 3′-UTR transcripts, which plays a major role in protein production on mTOR activation. Meanwhile, relatively smaller portion of the polysomes formed with long 3′-UTR transcripts, which minimally contributes to protein production. Thus, we conclude that the overexpression of selected E2 and E3 ligase complexes is due to mTOR-promoted 3′-UTR shortening of those mRNAs. In this study, we used genetically well-defined MEFs to investigate the molecular signatures of mTOR-activated transcriptome and discovered widespread 3′-UTR shortening due to dysregulated mTOR activation. Although a precise mechanism(s) of how mTOR activation leads to the 3′-UTR shortening in selected transcripts is unknown, we found that almost all known 3′-end processing factors alter their expression on changes in cellular mTOR activity in TSC1 −/− compared with WT MEFs, suggesting that mTOR-mediated 3′-UTR shortening occurs by multiple factors ( Supplementary Data 3 ). Analysis on pathways enriched in 3′-UTR-shortened transcripts and quantitative proteomics on mTOR activation identified ubiquitin-mediated proteolysis as an additional target pathway of mTOR. Considering the well-documented function of mTOR in the activation of cellular anabolic metabolism for rapid cell proliferation [33] , the newly discovered function of mTOR in ubiquitin-mediated proteolysis through 3′-UTR shortening is surprising. A recent study suggests a role of mTOR in the activation of proteasome through the modulation of a transcriptional network [21] . This study argued that the promotion of protein degradation pathway on mTOR activation is required for a continuous supply of amino acids to cellular systems, to maintain the steady-state protein synthesis. Our data set also indicates a marginal increase in the proteasome activity through a transcriptional upregulation of several proteasomal subunits ( Supplementary Fig. 4d ) and an increase in the polyubiquitination of proteins on mTOR activation ( Supplementary Fig. 4i ). Moreover, our data demonstrate that mTOR-promoted 3′-UTR shortening leads to the overexpression of selected E2 and E3 components in ubiquitin ligase complexes ( Figs 3b,d and 4b ), which is known to increase polyubiquitination of their substrates [34] , [35] , [36] , [37] , [38] , [39] , [40] . Therefore, it is possible that the enrichment of polyubiquitination in cellular proteins on mTOR activation could come from selective polyubiquitination of those E2 and E3 substrates. Together, our study proposes the molecular mechanism of how mTOR pathway selects proteins to degrade through 3′-UTR shortening of a subset of mRNAs. The E2 and E3 enzymes upregulated by mTOR-driven 3′-UTR shortening mostly target cell cycle regulators, tumour suppressors and pro-apoptotic proteins for ubiquitin–proteasome system [35] , [41] . For instance, Rbx1, Trip12 or Anapc1/5 are all components of E3 ligase complexes that selectively polyubiquitinate Arf and Cyclins, and Birc6 E3 ligase targets Caspase 3/7 for degradation [35] , [41] , [42] . For rapidly proliferating cells, a timely removal of cell cycle regulators such as Arf and Cyclins is a key step for rapid progression of the cell cycle [35] . Therefore, our findings are particularly important, because unlike a previous argument it explains how upregulated mTOR and consequent proteasome activation recycles proteins that are only needed to foster a cellular environment favourable to rapid cell proliferation. Thus, we suggest that this selective proteolysis not only provides a surplus of amino acids to cellular systems but also makes cells proliferate rapidly by efficient modulation of the cellular levels of cell cycle regulators. Although a consensus on the role of mTOR is an increase in global protein synthesis, many studies suggest that mTOR-modulated promotion of protein synthesis requires numerous trans - and cis -acting elements [16] . In particular, 5′TOP and 5′PRTE sequence features found in the 5′-UTR in a group of mRNAs render the activation of cellular pathways such as translation, cellular invasion and metastasis [17] , [18] . One of the distinctive behaviours of this group of mRNAs is their acute dissociation from actively translating polysomes in response to mTOR inhibition [17] , [18] . Interestingly, Rpl22 mRNA contains both 5′TOP and 3′-UTR-shortening molecular features. Compared with mRNAs containing 5′TOP feature, the formation of polysomes with this particular mRNA is not entirely dependent on 5′TOP but is rather regulated by 3′-UTR shortening, because the long 3′-UTR Rpl22 mRNA was not enriched in the polysome fractions in TSC1 −/− MEFs ( Supplementary Fig. 4a,c ). As most of the 3′-UTR-shortened transcripts for ubiquitin-mediated proteolysis do not contain mTOR-responsive sequence features in their 5′-UTR ( Supplementary Fig. 3d ), 3′-UTR shortening due to mTOR activation could function in protein synthesis independent of 5′-UTR structure of an mRNA and it presents an additional molecular signature targeted by the mTOR pathway. RNA-seq and alignments To evaluate transcriptome features under mTOR hyperactivation at nucleotide-wise resolution, we performed RNA-seq analysis of poly(A+) RNAs isolated from WT and TSC1 −/− MEFs. In total, 63,742,790 paired-end reads for WT and 74,251,891 paired-end reads for TSC1 −/− MEFs were produced from Hi-Seq pipeline with length of 50 bp of each end. The short reads were aligned to the mm10 reference genome by TopHat [43] , with up to two mismatches allowed. The unmapped reads were first trimmed to remove poly-A/T tails (repeats of [A/N]s or [T/N]s) from read ends/starts and then aligned to the reference genome. It is worth noting that we only retained the reads with at least 30 bp in both ends after trimming. Finally, 87.1% of short reads from WT and 87.5% of sequence reads from TSC1 −/− MEFs were mapped to the reference genome by TopHat for APA analysis in the study. ApA analysis To detect the potential alternative PAS of a transcript between WT and TSC1 −/− MEFs, we evaluated candidate PAS motifs (AATAAA, ATTAAA, AGTAAA, CATAAA, TATAAA, GATAAA, ACTAAA, AATACA, AATATA, AAGAAA, AATAGA, AATGAA, TTTAAA, AAAATA, TATATA, AGATAA, ATTACA, AGAATA) [44] , [45] in the 3′-UTR of the transcript by contrasting the short-read coverage up/downstream of the site across WT and TSC1 −/− samples with χ 2 -test. Specifically, we first scaned the 3′-UTR of a transcript (by mm10 annotation) to identify PAS motifs as candidates of alternative PAS. For each candidate PAS, we calculated the mean coverage upstream of the site (N and M) and downstream of the site (n and m) with (N, n) denoting the coverage in WT and (M, m) denoting the coverage in TSC1 −/− . In the calculation, the upstream region starts at the beginning of the last coding exon adjacent to the 3′-UTR of the transcript and ends at the beginning of the PAS motif site. Next, a canonical 2 × 2 χ 2 -test was applied to report a P -value for each candidate site. The candidate PAS with the most significant P -value ≤0.05 was considered for further analysis. It is noteworthy that the χ 2 -test will report shortening events in both WT (when N/n>M/m) and TSC1 −/− (when N/n<M/m). Out of the 5,160 transcripts, 846 (16.4%) show a P -value ≤0.05 in TSC1 −/− MEFs and 69 (1.3%) a show P -value ≤0.05 in WT MEFs. Scatter plot for differential expression and ApA analysis To select candidate transcripts with sufficient signal for reliable differential expression analysis and 3′-UTR-shortening identification, we first analysed the short-read alignments of the RNA-seq data against mouse mm10 reference genome using Cufflink [12] . In the alignments, 14,378 and 14,175 transcripts are considered ‘expressed’ in WT and TSC1 −/− cell lines, respectively, with a FPKM (fragments per kilobase of transcript per million mapped reads) cutoff=0.17. The union of the two sets gives 15,340 transcripts that are expressed in at least one of the cell lines. We further filtered out the transcripts with positional short-read coverage ≤25 in the entire 3′-UTR in both cell lines. In addition, transcripts with 3′-UTR overlapping exons in the strand in opposite direction were removed to avoid mingled short-read signals that might lead to inaccurate 3′-UTR-shortening identification. Finally, to allow precise PAS analysis, only transcripts with at least two occurrences of the 18 PAS motifs in the 3′-UTR are retained in the study. The entire pruning procedure left 5,160 transcripts for further analysis. Measurement of RSI A numerical presentation of 3′-UTR shortening was developed by calculating the RSI of a given transcript. A relative expression of total or longer 3′-UTR-containing transcripts was measured by normalizing to total amount of RNAs used in RT–qPCR analysis. The following equation was used to determine the RSI. LI=[normalized expression of longer 3′-UTR-containing transcript]/[normalized expression of total (long+short) transcript] RSI=−Log 2 (LI/[LI in reference cell line]); thus, RSI=0 for a reference cell line. If RSI >0 in a target cell line, then there is a 3′-UTR shortening. If RSI <0 in a target cell line, then there is a 3′-UTR lengthening. The RSI contains the information about the changes in the proportion of a longer 3′-UTR-containing transcript in a given cellular context compared with a reference cell. For example, a value of 1 in the RSI of a transcript indicates that the proportion of the longer 3′-UTR-containing transcript of the total (long+short) transcript decreases by 50% compared with that of the reference cell line, indicating an enrichment of 3′-UTR-shortened transcript (that is, 3′-UTR shortening). TMT labelling and proteomics analysis Total cell lysates of WT and TSC1 −/− MEFs were prepared by re-suspending the cells in 2% w/v SDS solution in 50 mM Tris pH 7.4 and heating to 95 °C for 5 min, followed by 5 passes through a 25-gauge needle. Cell debris was removed by centrifugation at 16,100 g for 10 min. The resulting proteins were quantified by BCA assay and 100 μg digested using the FASP protocol [46] . Peptides were cleaned up using Waters Sep-Pak SPE cartridges (WAT054925, Waters Corp., Milford, MA) and labelled using isobarically labelled TMT 6-plex reagents (9,0061, Thermo Scientific), following the manufacturer’s protocol. The labelled peptides were pooled and again cleaned up by Sep-Pak SPE. Peptides were fractionated by high-pH reversed-phase chromatography into 40 fractions and recombined to give 12 fractions for analysis by LC–electrospray ionization–MS/MS [47] . Approximately 1.0–1.5 μg of each recombined fraction was analysed on a Velos Orbitrap mass spectrometer using HCD dissociation as per Lin-Mosier et al. [48] . Three repeats of independent experiments were carried out for statistical confidence. Protein identification and quantification MS data were searched against a Uniprot mouse database (downloaded July 2013) containing common protein contaminants plus all reversed sequences (102,424 total sequences) using X!Tandem. Search parameters included semi-tryptic cleavage with one missed cleavage allowed, 0.01 Da monoisotopic precursor mass error, ±0.5 Da product mass error, fixed modifications of carbamidomethylation at C, TMT label at K and amino termini, and variable modification of oxidation at M and P. All search results were loaded into Scaffold Q+ (Proteome Software Inc.) as a Mudpit sample and filtered to 99% protein confidence, 95% peptide confidence with 6 p.p.m. precursor mass error, and 1 non-tryptic terminus and 2 peptides per protein resulting in 2,778 proteins identified at 0% protein and peptide false discovery rate (FDR). The fold change ratios were exported from Scaffold Q+ for further bioinformatic analysis. Western blotting and antibodies The following antibodies were used in this study; anti-mTOR (cat. 2,972, Cell Signaling, 1:500), anti-TSC1 (cat. 6,935, Cell Signaling, 1:500), anti-ACTIN (cat. A2668, Sigma, 1:2,000), anti-Phospho-S6 ribosomal protein (cat. 2211, Cell Signaling, 1:1,000), anti-UBIQUITIN (cat. 13–1600, Life technologies, 1:500), anti-Ube2b (cat. 4944, Cell Signaling, 1:1,000), anti-Ube2i (cat. 4786, Cell Signaling, 1:1,000), anti-Rbx1 (cat. 11922, Cell Signaling, 1:500) and anti-tubulin (cat. sc-53646, Santa Cruz Biotechnology, 1:2,000). Uncropped scans of western blotting are provided in Supplementary Figs 5–8 . Polysome isolation and analysis Isolation of polysome fractions from total cell lysates using sucrose gradient was carried out as previously described [3] . Briefly, cells were lysed in the polysome buffer (20 mM Tris pH 7.4, 150 mM NaCl, 5 mM MgCl 2 , 1 mM dithiothreitol, 100 μg ml −1 cycloheximide and 1% Triton X-100). Cell extracts were loaded onto sucrose gradient (5%–45%). Fractionation was done by centrifugation at 36,000 r.p.m. for 2 h at 4 °C. Eleven fractions were collected for the analysis. The percentage of mRNAs in each fraction was calculated as described previously [18] . Five per cent (v/v) of total RNAs in each fraction were used for RT–qPCR. Relative enrichment of total or long transcripts was measured by normalizing to BC200 RNA, which were added to each fraction for recovery and normalization control. The signals of total transcripts for a gene in all fractions of TSC1 −/− were combined and set as 100%. Next, the percentage of a total transcript in each fraction was calculated and the distribution of total transcripts for a gene was shown by the fraction. In case of long 3′-UTR transcripts, the signals of long transcripts in all fractions were combined and the relative amount of long transcripts was scaled down based on the relative differences between total and long transcript signals in input. The percentage and distribution of long transcripts in each fraction were calculated and presented. The same procedure was applied to the rest of transcripts (long and total in WT and TSC1 −/− treated with Torin1) by considering total transcripts in TSC1 −/− as 100%. How to cite this article: Chang, J. -W. et al. mRNA 3′-UTR shortening is a molecular signature of mTORC1 activation. Nat. Commun. 6:7218 doi: 10.1038/ncomms8218 (2015). Accession code. The accession number for the RNA-seq data in this study is SRP056624. The accession number for the proteome data in this study is PXD002006.